Tribbles 3 mediates endoplasmic reticulum stress-induced insulin resistance in skeletal muscle Endoplasmic reticulum stress has been linked to insulin resistance in multiple tissues but the role of endoplasmic reticulum stress in skeletal muscle has not been explored. Endoplasmic reticulum stress has been reported to increase tribbles 3 expression in multiple cell lines. Here, we report that high-fat feeding in mice, and obesity and type 2 diabetes in humans significantly increases tribbles 3 and endoplasmic reticulum stress markers in skeletal muscle. Overexpression of tribbles 3 in C2C12 myotubes and mouse tibialis anterior muscles significantly impairs insulin signalling. Incubation of C2C12 cells and mouse skeletal muscle with endoplasmic reticulum stressors thapsigargin and tunicamycin increases tribbles 3 and impairs insulin signalling and glucose uptake, effects reversed in cells overexpressing RNAi for tribbles 3 and in muscles from tribbles 3 knockout mice. Furthermore, tribbles 3 knockout mice are protected from high-fat diet-induced insulin resistance in skeletal muscle. These data demonstrate that tribbles 3 mediates endoplasmic reticulum stress-induced insulin resistance in skeletal muscle. While modern medicine has succeeded in reducing or eliminating many diseases, the incidence of type 2 diabetes continues to rise. Skeletal muscle is one of the major sites of glucose disposal in the body [1] . A major characteristic of patients with type 2 diabetes is reduced insulin sensitivity in skeletal muscle. Although considerable progress has been made in understanding skeletal muscle insulin resistance, the underlying mechanisms have not been fully elucidated. Tribbles 3 (TRB3), a mammalian homologue of Drosophila tribbles, is a pseudokinase and therefore contains a kinase domain without enzymatic activity [2] . TRB3 is expressed in various tissues, including liver, adipose tissue, heart and skeletal muscle [3] , [4] , [5] , [6] . Emerging data suggest that TRB3 has strikingly different metabolic functions depending on the tissue studied. In the liver, TRB3 binds and inhibits Akt activity, leading to impaired insulin signalling [3] . Overexpression of TRB3 in mouse liver results in decreased glycogen content, increased hepatic glucose output and blood glucose concentrations, and impaired glucose tolerance [3] , whereas disruption of TRB3 in mouse liver by RNAi improves glucose tolerance [7] . In pancreatic β cells, TRB3 expression increases with type 2 diabetes in mice and humans and the overexpression of TRB3 in mice inhibits glucose-stimulated insulin secretion and impairs glucose homoeostasis [8] . However, studies performed in adipose tissue suggest TRB3 has a very different role, functioning in the regulation of fatty acid oxidation through ubiquitination of acetyl-CoA carboxylase [4] . Mice overexpressing TRB3 in adipose tissue are protected from diet-induced obesity due to enhanced fatty acid oxidation [4] . There has been limited investigation on the role of TRB3 in skeletal muscle. Our study has shown that overexpression of TRB3 in C2C12 muscle cells inhibits insulin-stimulated Akt phosphorylation and decreases insulin-stimulated glucose uptake [6] . More recently, TRB3 expression has been shown to be elevated in skeletal muscle from patients with type 2 diabetes [9] . In another study, TRB3 expression was reported to be decreased in the skeletal muscle of ob/ob mice after a single bout of exercise, which has been implicated in post-exercise insulin sensitivity [10] . The endoplasmic reticulum (ER) is the major site in the cell for lipid and protein synthesis, folding, assembly and trafficking, as well as cellular Ca 2+ storage [11] , [12] . Interference with ER function by conditions such as high-fat feeding, virus infection and glucose deprivation are referred to as ER stress [12] , [13] , [14] . ER stress is characterized by increases in a number of transcription factors such as activating transcription factor 6 (ATF6), CCAAT/enhancer-binding protein homologous protein (CHOP) and X-box binding protein 1 (XBP1) and phosphorylation of protein kinase-like ER kinase (PERK), leading to translational attenuation and cell cycle arrest [12] , [13] , [14] . In the liver, ER stress has also been shown to cause c-Jun N-terminal kinase (JNK) activation, which results in increased IRS1 serine phosphorylation and subsequent insulin resistance [15] , whereas inhibition of ER stress by chemical chaperones protects high-fat-fed mice from insulin resistance [16] . In pancreatic β cells, high glucose [17] , [18] , free fatty acids [19] , [20] and inflammatory cytokines [21] cause ER stress, which has emerged as a key player for β-cell dysfunction and death during the progression of type 1, type 2 and genetic forms of diabetes. In the kidney, mice with a heterozygous constitutive knockin mutation of a mutant-binding immunoglobulin protein (BiP) have evidence of ER stress, associated with age-related renal tubular atrophy, interstitial fibrosis and glomerulosclerosis [22] . ER stress also occurs in cardiac myocytes and cardiac tissue in response to various stressors, including ischaemia, inflammation and exposure to alcohol, which has been associated with cardiomyopathy and apoptosis [23] , [24] , [25] . Although the effects of ER stress in multiple tissues have been established, the role of ER stress in skeletal muscle is poorly understood. However, several conditions have recently been suggested to cause ER stress in skeletal muscle, including type 1 diabetes [26] , high-fat feeding [27] , overexpression of stearoyl-CoA desaturase 1 ( [28] ) and exercise [29] . In the current study, we tested the hypothesis that TRB3 mediates ER stress-induced insulin resistance in skeletal muscle. We find that ER stress in both C2C12 muscle cells in culture and adult mouse skeletal muscle increases TRB3 expression. Overexpression of TRB3 in C2C12 myotubes and adult mouse skeletal muscle in vivo inhibits insulin signalling and glucose uptake. ER stress-induced insulin resistance is reversed with knockdown of TRB3 in C2C12 myotubes and in skeletal muscle of TRB3 knockout mice. In addition, TRB3 knockout mice are protected from high-fat diet-induced insulin resistance. These data demonstrate that TRB3 mediates ER stress-induced insulin resistance in skeletal muscle. Obesity and diabetes increase TRB3 in skeletal muscles TRB3 is expressed in multiple tissues, including liver, adipose tissue and pancreatic β cells [3] , [4] , [8] , and here we first determined the mRNA expression profile of TRB3 in multiple mouse skeletal muscles. TRB3 mRNA expression was lower in the white gastrocnemius muscle (WG) and higher in other muscles, including tibialis anterior (TA), red gastrocnemius (RG), soleus (Sol) and extensor digitorum longus (EDL) muscles ( Fig. 1a ). To determine if altered metabolic states affect TRB3 expression in mouse skeletal muscle, mice were fed a high-fat diet for 6 weeks. This treatment increased body weight, blood glucose and serum insulin concentrations ( Supplementary Fig. S1 ), and significantly increased TRB3 mRNA expression in TA muscles by 5.2-fold ( Fig. 1b ). To determine the effects of insulin and fatty acids on the regulation of TRB3, C2C12 myotubes were studied. Insulin incubation at 10 nM and 100 nM for 16 h increased TRB3 expression by 4.2- and 5.3-fold, respectively ( Fig. 1c ), whereas palmitate incubation at 0.75 mM, a physiological dosage [30] , increased TRB3 expression by 1.7-fold ( Fig. 1d ). Incubation of C2C12 myotubes with insulin and palmitate increased mRNA expression of ER stress markers GRP78 and CHOP, and the increase was abrogated by chemical inhibitors for insulin signalling molecules and chemical chaperones (4-phenyl butyric acid and dimethyl sulphoxide) ( Fig. 1e ). 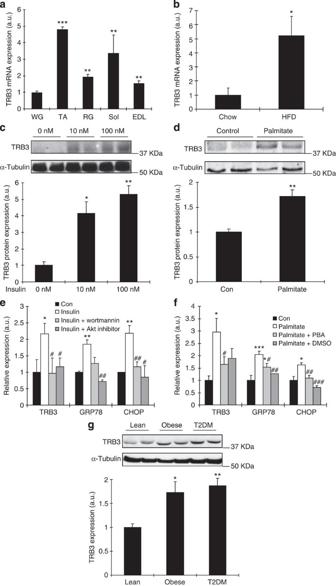Figure 1: Regulation of TRB3 expression in C2C12 cells and mouse skeletal muscle. (a) Female ICR mice (12 weeks old) were killed by cervical dislocation and white gastrocnemius (WG), tibialis anterior (TA), red gastrocnemius (RG), soleus (Sol) and extensor digitorum longus (EDL) muscles were dissected and frozen. Real-time PCR was performed to determine mRNA expression of TRB3 in multiple muscles (n=3). (b) Male C57BL/6 mice (8 weeks old) were fed a high-fat diet for 6 weeks. TA muscle was dissected to determine mRNA expression of TRB3 (n=6). (c–f) C2C12 cells were differentiated for 6 days and incubated with 0, 10 or 100 nM of insulin (c); 0 or 0.75 mM palmitate (d) with 2% BSA for 16 h, and protein extracts were used for western blot analysis to determine TRB3 expression as described in Methods (n=4). Additional myotubes were preincubated with DMSO (0.1% v/v), PI3 kinase inhibitor (100 nM; Wortmannin from Sigma) or Akt inhibitor (10 μM; Akt inhibitor VIII from EMD) 30 min before incubation with 0 or 100 nM of insulin (e); with chemical chaperones (5 mM; 4-phenyl butyric acid, PBA from Sigma or 0.5% v/v: DMSO) 30 min before incubation with 0 or 0.75 mM palmitate (f) for 16 h to determine mRNA expression of TRB3, GRP78 and CHOP (n=3). (g) TRB3 western blot analysis of vastus lateralis muscle from lean, obese or diabetic subjects (n=6–13). Data are the means±s.e.m. * indicatesP<0.05, ** indicatesP<0.01 and *** indicatesP<0.001 versus WG muscle or control. # indicatesP<0.05, ## indicatesP<0.01 and ### indicatesP<0.001 versus corresponding control, using one-way ANOVA (a,c,g), Student’st-test (b,d) and two-way ANOVA with Bonferroni correction (e,f). Figure 1: Regulation of TRB3 expression in C2C12 cells and mouse skeletal muscle. ( a ) Female ICR mice (12 weeks old) were killed by cervical dislocation and white gastrocnemius (WG), tibialis anterior (TA), red gastrocnemius (RG), soleus (Sol) and extensor digitorum longus (EDL) muscles were dissected and frozen. Real-time PCR was performed to determine mRNA expression of TRB3 in multiple muscles ( n =3). ( b ) Male C57BL/6 mice (8 weeks old) were fed a high-fat diet for 6 weeks. TA muscle was dissected to determine mRNA expression of TRB3 ( n =6). ( c – f ) C2C12 cells were differentiated for 6 days and incubated with 0, 10 or 100 nM of insulin ( c ); 0 or 0.75 mM palmitate ( d ) with 2% BSA for 16 h, and protein extracts were used for western blot analysis to determine TRB3 expression as described in Methods ( n =4). Additional myotubes were preincubated with DMSO (0.1% v/v), PI3 kinase inhibitor (100 nM; Wortmannin from Sigma) or Akt inhibitor (10 μM; Akt inhibitor VIII from EMD) 30 min before incubation with 0 or 100 nM of insulin ( e ); with chemical chaperones (5 mM; 4-phenyl butyric acid, PBA from Sigma or 0.5% v/v: DMSO) 30 min before incubation with 0 or 0.75 mM palmitate ( f ) for 16 h to determine mRNA expression of TRB3, GRP78 and CHOP ( n =3). ( g ) TRB3 western blot analysis of vastus lateralis muscle from lean, obese or diabetic subjects ( n =6–13). Data are the means±s.e.m. * indicates P <0.05, ** indicates P <0.01 and *** indicates P <0.001 versus WG muscle or control. # indicates P <0.05, ## indicates P <0.01 and ### indicates P <0.001 versus corresponding control, using one-way ANOVA ( a , c , g ), Student’s t -test ( b , d ) and two-way ANOVA with Bonferroni correction ( e , f ). Full size image Given that obesity and type 2 diabetes are characterized by impaired metabolic states, we hypothesized that skeletal muscle from human patients with these diseases would have increased TRB3 expression. Compared with age- and sex-matched controls, TRB3 expression was significantly higher in the vastus lateralis muscle of subjects with obesity and type 2 diabetes ( Fig. 1g ). Taken together, all of these studies demonstrate that multiple metabolic perturbations regulate TRB3 expression in both mouse and human skeletal muscle. TRB3 inhibits insulin signalling in vitro and in vivo Given that TRB3 was increased with altered metabolic states, we next determined if overexpression of TRB3 would impair insulin signalling. We have previously shown that overexpression of TRB3 in C2C12 cells decreases insulin-stimulated Akt activity via direct binding to Akt [6] . To determine if this effect was specific for Akt or has a more generalized effect on insulin signalling, we infected C2C12 myotubes with adenovirus containing either GFP control or TRB3. Overexpression of TRB3 did not affect tyrosine phosphorylation of the insulin receptor and IRS2 ( Fig. 2a ; Supplementary Fig. S2 ). In contrast, compared with control cells expressing GFP, overexpression of TRB3 resulted in a significant decrease in both submaximal and maximal insulin-stimulated IRS1 Tyr 612 phosphorylation ( Fig. 2b ), an upstream regulator of PI3 kinase activity [31] . 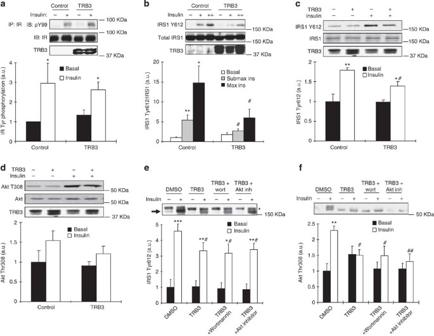Figure 2: Effects of TRB3 on insulin signalling in C2C12 cells and mouse skeletal muscle. (a) Coimmunoprecipitation experiments were performed on C2C12 cells overexpressed with TRB3. Insulin receptor (IR) immunoprecipitates (IP) were immunoblotted with phospho-tyrosine specific antibody (pY99). Immunoblotting (IB) with IR-specific antibody confirmed equal protein (n=3). (b) IRS1 Tyr612 phosphorylation with TRB3 overexpression was determined in the C2C12 cells incubated with submaximal insulin (2.7 nM) or maximal insulin (100 nM) (n=5). (c,d) TRB3 was overexpressed in female ICR mouse (10 weeks old) TA muscle by a direct DNA injection followed by electroporation. At 2 weeks after electroporation, mice were killed 10 min after injection of either saline (basal) or 1 U per kg body weight of IP insulin. TA muscles were collected, frozen, and processed for Western blot analysis to determine phosphorylation of IRS1 Tyr612 (c) and Akt Thr308 (d) (n=6). (e,f) C2C12 myotubes were preincubated with DMSO, PI3 kinase inhibitor (100 nM; wortmannin from Sigma) or Akt inhibitor (10 μM; Akt inhibitor VIII from EMD) 30 min before infection with TRB3. Lysates were subjected to gel electrophoresis to determine the IRS1 tyrosine phosphorylation at 612 (e; arrow indicates the IRS1 Tyr612 and asterisk indicates non-specific band) and Akt threonine phosphorylation at 308 (n=3). Data are the means±s.e.m. * indicatesP<0.05, ** indicatesP<0.01, and *** indicatesP<0.001 versus basal in the same group. # indicatesP<0.05 and ## indicatesP<0.01 versus corresponding control, using two-way ANOVA with Bonferroni correction. Figure 2: Effects of TRB3 on insulin signalling in C2C12 cells and mouse skeletal muscle. ( a ) Coimmunoprecipitation experiments were performed on C2C12 cells overexpressed with TRB3. Insulin receptor (IR) immunoprecipitates (IP) were immunoblotted with phospho-tyrosine specific antibody (pY99). Immunoblotting (IB) with IR-specific antibody confirmed equal protein ( n =3). ( b ) IRS1 Tyr612 phosphorylation with TRB3 overexpression was determined in the C2C12 cells incubated with submaximal insulin (2.7 nM) or maximal insulin (100 nM) ( n =5). ( c , d ) TRB3 was overexpressed in female ICR mouse (10 weeks old) TA muscle by a direct DNA injection followed by electroporation. At 2 weeks after electroporation, mice were killed 10 min after injection of either saline (basal) or 1 U per kg body weight of IP insulin. TA muscles were collected, frozen, and processed for Western blot analysis to determine phosphorylation of IRS1 Tyr612 ( c ) and Akt Thr308 ( d ) ( n =6). ( e , f ) C2C12 myotubes were preincubated with DMSO, PI3 kinase inhibitor (100 nM; wortmannin from Sigma) or Akt inhibitor (10 μM; Akt inhibitor VIII from EMD) 30 min before infection with TRB3. Lysates were subjected to gel electrophoresis to determine the IRS1 tyrosine phosphorylation at 612 ( e ; arrow indicates the IRS1 Tyr612 and asterisk indicates non-specific band) and Akt threonine phosphorylation at 308 ( n =3). Data are the means±s.e.m. * indicates P <0.05, ** indicates P <0.01, and *** indicates P <0.001 versus basal in the same group. # indicates P <0.05 and ## indicates P <0.01 versus corresponding control, using two-way ANOVA with Bonferroni correction. Full size image We next tested if TRB3 inhibits insulin signalling in adult mouse skeletal muscle. Overexpression of TRB3 (4-fold) in TA muscles by direct DNA injection significantly inhibited insulin-stimulated IRS1 Tyr 612 phosphorylation compared with empty vector-injected muscles ( Fig. 2c ), whereas insulin-stimulated Akt Thr 308 and Akt Ser 473 phosphorylation tended to decrease with TRB3 overexpression ( Fig. 2d and Supplementary Fig. S3 ). There was no effect of TRB3 overexpression on total expression of IRS1 and Akt ( Fig. 2c ). These data suggest that overexpression of TRB3 impairs proximal insulin signalling in skeletal muscle. To determine the mechanism by which TRB3 regulates IRS1 signalling, we overexpressed Flag-TRB3 in 293 cells and found an association of TRB3 with IRS1 by both immunoprecipitation-Flag/immunoblotting-IRS1 and immunoprecipitation-IRS1/immunoblotting-Flag ( Supplementary Fig. S4a,b ). To examine if TRB3-IRS1 binding is present in skeletal muscle, we used TA muscle lysates overexpressing Flag-tagged TRB3. Lysates were immunoprecipitated with either IgG or IRS1 antibodies and immunoblotted with Flag to detect TRB3. The association was only present in the muscle lysates immunoprecipitated with IRS1 antibody but not in lysates immunoprecipitated with IgG ( Supplementary Fig. S4c ), suggesting that TRB3 binds to IRS1 in mouse skeletal muscle. Taken together with our previous study showing Akt binding to TRB3 in muscle [6] , these data suggest that TRB3 inhibits IRS1 and Akt signalling presumably by direct or indirect association with these proteins. We next overexpressed TRB3 and inhibited IRS1 downstream signalling proteins PI3K and Akt using chemical inhibitors, wortmannin and Akt inhibitor VIII, to test the hypothesis if the effect of TRB3 on IRS1 and Akt phosphorylation is due to decreased Akt and downstream signalling molecules, which in turn feedback to inhibit IRS1, and found that the effect of TRB3 to impair IRS1 and Akt phosphorylation was not altered by the inhibitors ( Fig. 2e ), suggesting that the effect was not due to feedback inhibition of IRS1 and Akt. Obesity and diabetes increase ER stress in skeletal muscle Based on our current data showing that overexpression of TRB3 impaired insulin signalling and a previous study showing the induction of TRB3 by ER stress through ATF4-CHOP pathway in multiple cell lines [32] , we hypothesized that TRB3 may mediate ER stress-induced insulin resistance in skeletal muscle. Therefore, we determined if high-fat feeding increased ER stress markers. Indeed, high-fat diet for 6 weeks increased expression of ER stress marker proteins including XBP1, CHOP and BiP ( Fig. 3a ), consistent with a previous study showing high-fat feeding of mice increasing mRNA expression of ER stress markers in skeletal muscle [27] . Phosphorylation of inositol-requiring enzyme 1 alpha (IRE1α) at Ser 724 and JNK was not altered by high-fat feeding ( Fig. 3a ). Next, we measured markers of ER stress in muscle biopsies of the human patients, and found that the obesity- and diabetes-induced increases in TRB3 were accompanied by a significant elevation of several ER stress markers ( Fig. 3b ). The expression of XBP1 and CHOP was significantly elevated in patients with diabetes, while there was a tendency towards an increase in these markers in obese patients ( Fig. 3c ). Expression of BiP was significantly elevated in patients with both obesity and diabetes ( Fig. 3e ). The phosphorylation of IRE1α was not altered ( Fig. 3f ). In addition, JNK expression and phosphorylation were also not altered in the obese or diabetic patients ( Fig. 3g ). The expression of TRB3 and XBP1 was significantly correlated with body mass index, and TRB3 expression was also correlated with XBP1 ( Supplementary Fig. S5 ). Thus, obesity and type 2 diabetes increase several, but not all, ER stress markers in human skeletal muscle, and expression of several ER stress markers is correlated with body mass index (BMI). 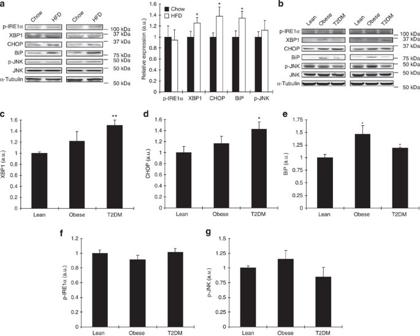Figure 3: Expression of ER stress markers in mouse and human skeletal muscle. (a) TA muscle lysates from high-fat-fed mice were used to determine the expression of ER stress markers by western blot analysis (n=6). (b–g) Western blot analysis was done to measure proteins involved in ER stress in vastus lateralis muscle from lean, obese or diabetic subjects (n=6–13). Data are the means±s.e.m. * indicatesP<0.05 and ** indicatesP<0.01 versus chow or lean controls, using Student’st-test (a) and one-way ANOVA. Figure 3: Expression of ER stress markers in mouse and human skeletal muscle. ( a ) TA muscle lysates from high-fat-fed mice were used to determine the expression of ER stress markers by western blot analysis ( n =6). ( b – g ) Western blot analysis was done to measure proteins involved in ER stress in vastus lateralis muscle from lean, obese or diabetic subjects ( n =6–13). Data are the means±s.e.m. * indicates P <0.05 and ** indicates P <0.01 versus chow or lean controls, using Student’s t -test ( a ) and one-way ANOVA. Full size image ER stress induces TRB3 and inhibits insulin signalling On the basis of our current data showing that overexpression of TRB3 impaired insulin signalling and that elevations of TRB3 were associated with increased ER stress markers, we next used C2C12 cells to test the hypothesis that TRB3 mediates ER stress-induced insulin resistance in skeletal muscle. TRB3 protein was barely detected in C2C12 cells under basal conditions and after 1 h of thapsigargin treatment, an ER stressor. However, 2–4 h of thapsigargin treatment significantly increased TRB3 expression ( Supplementary Fig. S6 ). Incubation of C2C12 cells with an additional ER stressor, tunicamycin, also resulted in a robust increase in TRB3 expression, similar to thapsigargin ( Fig. 4a ). To investigate the effects of these ER stressors on insulin signalling, C2C12 cells were incubated with tunicamycin and thapsigargin for 4 h, followed by maximal insulin stimulation for 15 min. Tunicamycin significantly impaired insulin-stimulated IRS1 Tyr 612 and Akt Thr 308 phosphorylation by 67% and 27%, respectively ( Fig. 4c ). Thapsigargin also inhibited insulin-stimulated phosphorylation of IRS1 and Akt ( Supplementary Fig. S7 ). These data demonstrate that ER stressors induce TRB3 expression and impair insulin signalling in C2C12 cells. 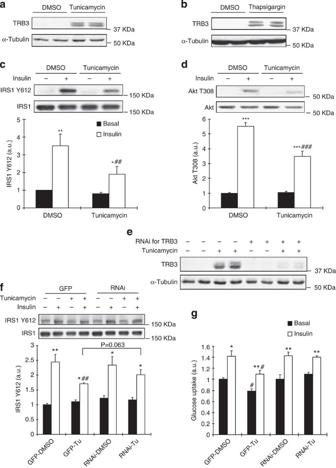Figure 4: Effects of ER stress and TRB3 in insulin signalling and glucose uptake in C2C12 cells. (a,b) C2C12 myotubes were incubated with ER stressors, tunicamycin (1 μg ml−1;a) or thapsigargin (1.3 μg ml−1;b), for 4 h. Lysates were subjected to western blot analysis to determine TRB3 expression. (c,d) C2C12 myotubes were incubated with tunicamycin for 4 h followed by 100 nM of insulin for 10 min. Insulin-stimulated IRS1 tyrosine phosphorylation at 612 (c) and Akt phosphorylation at threonine 308 (d) were determined by western blot analysis (n=4). (e–g) C2C12 myotubes were infected with adenovirus containing RNAi for TRB3. (e) ER stress-induced TRB3 expression was determined by western blot analysis. Cells were incubated in the presence or absence of tunicamycin to determine IRS1 Tyr612 phosphorylation (f) and glucose uptake (g) upon insulin stimulation (100 nM) (n=6). Data are the means±s.e.m. * indicatesP<0.05, ** indicatesP<0.01 and *** indicatesP<0.001 versus basal in the same group. # indicatesP<0.05, ## indicatesP<0.01 and ### indicatesP<0.001 versus corresponding control, using two-way ANOVA with Bonferroni correction. Figure 4: Effects of ER stress and TRB3 in insulin signalling and glucose uptake in C2C12 cells. ( a , b ) C2C12 myotubes were incubated with ER stressors, tunicamycin (1 μg ml −1 ; a ) or thapsigargin (1.3 μg ml −1 ; b ), for 4 h. Lysates were subjected to western blot analysis to determine TRB3 expression. ( c , d ) C2C12 myotubes were incubated with tunicamycin for 4 h followed by 100 nM of insulin for 10 min. Insulin-stimulated IRS1 tyrosine phosphorylation at 612 ( c ) and Akt phosphorylation at threonine 308 ( d ) were determined by western blot analysis ( n =4). ( e – g ) C2C12 myotubes were infected with adenovirus containing RNAi for TRB3. ( e ) ER stress-induced TRB3 expression was determined by western blot analysis. Cells were incubated in the presence or absence of tunicamycin to determine IRS1 Tyr612 phosphorylation ( f ) and glucose uptake ( g ) upon insulin stimulation (100 nM) ( n =6). Data are the means±s.e.m. * indicates P <0.05, ** indicates P <0.01 and *** indicates P <0.001 versus basal in the same group. # indicates P <0.05, ## indicates P <0.01 and ### indicates P <0.001 versus corresponding control, using two-way ANOVA with Bonferroni correction. Full size image To test the hypothesis that TRB3 mediates ER stress-induced alterations in insulin signalling and glucose uptake, we performed knockdown (80%) studies of TRB3 in C2C12 cells and incubated the cells with tunicamycin for 4 h. Tunicamycin treatment increased TRB3 and this effect was significantly blunted by RNAi ( Fig. 4e ). Tunicamycin treatment impaired insulin-stimulated IRS1 Tyr 612 phosphorylation, and this impairment was partially rescued by knockdown of TRB3 ( Fig. 4f ). In parallel, tunicamycin impaired basal and insulin-stimulated glucose uptake, an effect that was completely rescued by TRB3 knockdown ( Fig. 4g ). GLUT4 expression was not changed in all groups ( Supplementary Fig. S8 ). These data demonstrate that TRB3 has an important role in ER stress-induced impairment in insulin signalling and glucose uptake in C2C12 cells. ER stress decreases glucose uptake via TRB3 in vivo Isolated EDL muscles were incubated with vehicle, tunicamycin or thapsigargin for 4 h, which resulted in a 4- and 3.3-fold increase in TRB3 mRNA expression, respectively ( Fig. 5a ). Tunicamycin and thapsigargin incubation also caused an increase in gene expression of ER stress markers BiP and CHOP ( Supplementary Fig. S9a,b ). Moreover, tunicamycin and thapsigargin treatment in EDL muscles significantly impaired insulin-stimulated glucose uptake ( Fig. 5b ) without changes in GLUT1 and GLUT4 expression ( Supplementary Fig. S9c,d ). These data suggest that ER stress induces expression of TRB3 and impairs insulin-stimulated glucose uptake in mouse skeletal muscle. 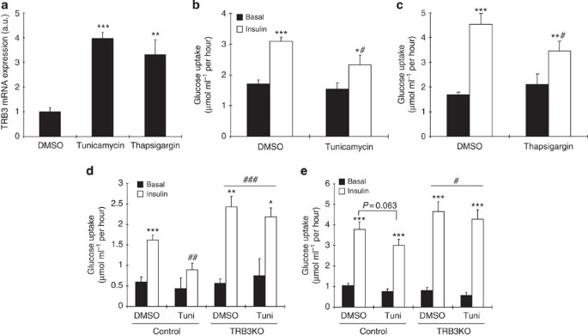Figure 5: ER stress and TRB3 inhibit glucose uptake in mouse skeletal muscle. (a–c) Extensor digitorum longus (EDL) muscles were dissected and incubated in the presence or absence of ER stressors, tunicamycin (1 μg ml−1) and thapsigargin (1.3 μg ml−1), for 4 h. After the incubation, EDL muscles were collected and used for mRNA measurement for TRB3 (a) (n=5). Insulin-stimulated glucose uptake from EDL with tunicamycin (b) and thapsigargin (c) was determined as described in Methods (n=5). (d,e) EDL (d) and Sol (e) muscles from wild type and TRB3KO mice were dissected and incubated with tunicamycin (1 μg ml−1) for 4 h (n=6–8). Data are the means±s.e.m. * indicatesP<0.05, ** indicatesP<0.01 and *** indicatesP<0.001 versus basal in the same group. # indicatesP<0.05, ## indicatesP<0.01, and ### indicatesP<0.001 versus corresponding control, using one-way ANOVA (a) and two-way ANOVA with Bonferroni correction. Figure 5: ER stress and TRB3 inhibit glucose uptake in mouse skeletal muscle. ( a – c ) Extensor digitorum longus (EDL) muscles were dissected and incubated in the presence or absence of ER stressors, tunicamycin (1 μg ml −1 ) and thapsigargin (1.3 μg ml −1 ), for 4 h. After the incubation, EDL muscles were collected and used for mRNA measurement for TRB3 (a) (n=5). Insulin-stimulated glucose uptake from EDL with tunicamycin ( b ) and thapsigargin ( c ) was determined as described in Methods ( n =5). ( d , e ) EDL ( d ) and Sol ( e ) muscles from wild type and TRB3KO mice were dissected and incubated with tunicamycin (1 μg ml −1 ) for 4 h ( n =6–8). Data are the means±s.e.m. * indicates P <0.05, ** indicates P <0.01 and *** indicates P <0.001 versus basal in the same group. # indicates P <0.05, ## indicates P <0.01, and ### indicates P <0.001 versus corresponding control, using one-way ANOVA ( a ) and two-way ANOVA with Bonferroni correction. Full size image We next used whole-body TRB3 knockout mice to determine if deletion of TRB3 rescued skeletal muscle from ER stress-induced insulin resistance. EDL and Sol muscles were isolated and incubated with vehicle or tunicamycin for 4 h. Tunicamycin impaired insulin-stimulated glucose uptake in control mice, and this effect was fully reversed in the TRB3KO mice ( Fig. 5d ). The TRB3KO mice also displayed elevated insulin-stimulated glucose uptake in the absence of tunicamycin ( Fig. 5d ). Taken together, these data demonstrate that ER stress impairs glucose uptake in mouse skeletal muscle and TRB3 mediates the development of insulin resistance by ER stressors. TRB3KO mice show no high-fat diet-induced insulin resistance Previous work has shown that 8 weeks old whole-body TRB3 knockout mice have normal glucose homoeostasis as evidenced by normal glucose and insulin tolerance, serum glucose, insulin, lipid levels and energy metabolism [33] . Consistent with these results, we also found that TRB3 knockout mice had normal body weights, fasting blood glucose concentrations and glucose tolerance at 26 weeks of age ( Supplementary Fig. S10 ). However, given that ER stress-induced insulin-stimulated glucose uptake was blunted in TRB3 knockout mice ( Fig. 5d ) and that high-fat feeding causes an increase in ER stress markers ( Fig. 3 ) [27] , we hypothesized that TRB3 knockout mice would be protected from high-fat diet-induced insulin resistance. To test this hypothesis, wild type and TRB3 knockout mice were fed a high-fat diet (HFD; 60% fat by kcal) for 8 weeks beginning at 6 weeks of age ( Supplementary Fig. S11a,b ). Food intake was not different between the groups (WT; 3.2±0.8 g per day versus TRB3KO; 2.9±0.9 g per day, mean±s.e.m.). Eight weeks of high-fat feeding increased body weights in both groups, but TRB3 knockout mice exhibited an 11% lower body weight compared with wild-type mice ( Fig. 6a ). TRB3 knockout mice had significantly better glucose tolerance than their control littermates ( Fig. 6b ), with a 35% decrease in glucose area under the curve ( Fig. 6c ). In the fasted state, serum concentrations of glucose, insulin and cholesterol were significantly lower in TRB3 knockout mice compared with wild-type mice, whereas free fatty acids and triglycerides concentrations were not different ( Supplementary Table S1 ). Serum adiponectin was significantly higher in the TRB3 knockout mice compared with wild type and leptin concentrations were lower ( Supplementary Table S1 ). 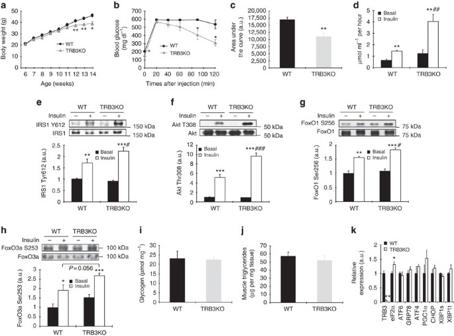Figure 6: Metabolic consequences of a high-fat diet in TRB3 knockout mice. (a–k) Wild type (WT) and TRB3 knockout mice at 6 weeks of age were placed on a high-fat diet for 8 weeks. (a) Body weights of male mice were tracked every week for 8 weeks during the high-fat diet. The TRB3 knockout mice showed lower body weight compared with wild-type mice. (b,c) Mice were fasted for 14 h to perform glucose tolerance test. The TRB3 knockout mice had lower fasting blood glucose concentration (b), improved glucose tolerance (b) and lower area under the curve during the glucose tolerance test (c). (d–k) Mice were fasted for 14 h and killed to determine insulin-stimulated glucose uptake from Sol muscles (d), insulin-stimulated phosphorylation of IRS1 (e), Akt (f), FoxO1 (g) and FoxO3a (h) in EDL muscles, and glycogen in TA muscles (i), triglycerides from gastrocnemius muscles (j) and mRNA expression of ER stress markers from TA muscles (k). Data are the means±s.e.m.,n=3–6 per group. * indicatesP<0.05, ** indicatesP<0.01 and *** indicatesP<0.001 versus wild type or basal in the same group. # indicatesP<0.05, ## indicatesP<0.01 and ### indicatesP<0.001 versus corresponding control in the wild type, using Student’st-test (a–c,k) and two-way ANOVA with Bonferroni correction (d–h). Figure 6: Metabolic consequences of a high-fat diet in TRB3 knockout mice. ( a – k ) Wild type (WT) and TRB3 knockout mice at 6 weeks of age were placed on a high-fat diet for 8 weeks. ( a ) Body weights of male mice were tracked every week for 8 weeks during the high-fat diet. The TRB3 knockout mice showed lower body weight compared with wild-type mice. ( b , c ) Mice were fasted for 14 h to perform glucose tolerance test. The TRB3 knockout mice had lower fasting blood glucose concentration ( b ), improved glucose tolerance ( b ) and lower area under the curve during the glucose tolerance test ( c ). ( d – k ) Mice were fasted for 14 h and killed to determine insulin-stimulated glucose uptake from Sol muscles ( d ), insulin-stimulated phosphorylation of IRS1 ( e ), Akt ( f ), FoxO1 ( g ) and FoxO3a ( h ) in EDL muscles, and glycogen in TA muscles ( i ), triglycerides from gastrocnemius muscles ( j ) and mRNA expression of ER stress markers from TA muscles ( k ). Data are the means±s.e.m., n =3–6 per group. * indicates P <0.05, ** indicates P <0.01 and *** indicates P <0.001 versus wild type or basal in the same group. # indicates P <0.05, ## indicates P <0.01 and ### indicates P <0.001 versus corresponding control in the wild type, using Student’s t -test ( a – c , k ) and two-way ANOVA with Bonferroni correction ( d – h ). Full size image To determine if the improved glucose tolerance is due to increased glucose uptake in skeletal muscle, we isolated Sol muscles from wild type and TRB3KO mice. Consistent with the improved glucose tolerance, insulin-stimulated glucose uptake was 2.8-fold higher in the muscles from TRB3KO mice ( Fig. 6d ). The increased glucose uptake was associated with increased insulin-stimulated IRS1 Tyr 612 , Akt Thr 308 and FoxO phosphorylation in TRB3KO mice ( Fig. 6e–h ). There was no difference in GLUT1 and GLUT4 expression ( Supplementary Fig. S11c,d ). The increases in insulin signalling and glucose uptake were not due to differences in muscle glycogen or triglycerides concentrations in the TRB3 knockout mice ( Fig. 6i ; Supplementary Fig. S11e ). TRB3 knockout mice did not have altered expression of ER stress markers in the muscle ( Fig. 6k ), consistent with ER stress regulation of TRB3 expression, and not TRB3 regulating ER stress markers. To further understand the mechanism for the improved glucose tolerance in the TRB3 knockout mice, we studied epididymal adipose tissue and liver. There was no difference in epididymal fat pad weight between wild type and TRB3 knockout mice ( Fig. 7a ). In contrast, tissue weights and triglyceride concentrations were significantly lower in the livers from TRB3 knockout mice ( Fig. 7b ), indicating that the TRB3 knockout mice were protected from high-fat diet-induced liver steatosis. Consistent with results in skeletal muscle, mRNA expression of ER stress markers in the liver were not different in TRB3 knockout mice compared with wild type ( Fig. 7d ). Analysis of mRNA expression of genes involved in glucose production (chREBP, PEPCK, G6PC, FBP1 and GCK) revealed similar levels of expression, whereas the genes involved in lipid synthesis (SREBP1, FAS, ACC and SCD1) were significantly lower in TRB3 knockout mice ( Fig. 7e ). The reduced expression of lipogenic enzymes is a likely mechanism for the decreased hepatosteatosis in high-fat-fed TRB3 knockout mice. Thus, the improved whole-body glucose homoeostasis in TRB3 knockout mice is likely due to changes in both skeletal muscle and liver. 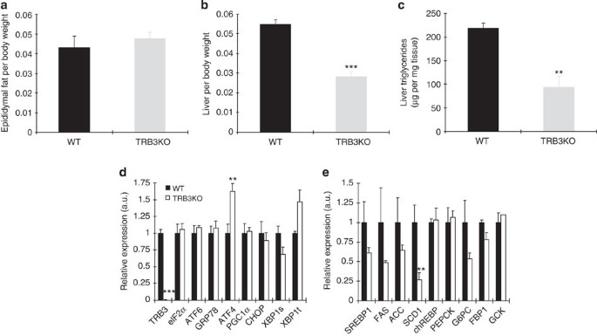Figure 7: The effects of TRB3 knockout on liver and adipose tissue in response to high-fat diet. Eight weeks after high-fat diet, wild type and TRB3 knockout mice were killed and epididymal fat (a) and liver (b) weights were determined. (c) Hepatic triglycerides were measured to determine liver steatosis. RNA was isolated from liver tissue to determine gene expression involved in ER stress (d) and lipogenesis and gluconeogenesis (e). Data are the means±s.e.m.,n=3–6 per group. ** indicatesP<0.01 and *** indicatesP<0.001 versus wild type, using Student’st-test. Figure 7: The effects of TRB3 knockout on liver and adipose tissue in response to high-fat diet. Eight weeks after high-fat diet, wild type and TRB3 knockout mice were killed and epididymal fat ( a ) and liver ( b ) weights were determined. ( c ) Hepatic triglycerides were measured to determine liver steatosis. RNA was isolated from liver tissue to determine gene expression involved in ER stress ( d ) and lipogenesis and gluconeogenesis ( e ). Data are the means±s.e.m., n =3–6 per group. ** indicates P <0.01 and *** indicates P <0.001 versus wild type, using Student’s t -test. Full size image Patients with type 2 diabetes are typically characterized by insulin resistance in skeletal muscle, the tissue responsible for the majority of insulin-stimulated glucose disposal [1] . Therefore, it is important to understand the molecular mechanisms leading to the development of skeletal muscle insulin resistance. In the current study, we tested the hypothesis that TRB3 has a role in ER stress-induced insulin resistance in skeletal muscle. The current results support this hypothesis as indicated by: 1) expression of TRB3 and ER stress markers was increased in multiple models of insulin resistance in muscle cells, mouse skeletal muscle and human skeletal muscle; 2) overexpression of TRB3 in C2C12 cells and skeletal muscle impaired insulin signalling and glucose uptake; 3) knockdown of TRB3 in C2C12 myotube and mouse models significantly blunted the effects of ER stressors to impair insulin signalling and glucose uptake; and 4) TRB3 knockout mice were protected from high-fat diet-induced insulin resistance. Our findings that TRB3 mediates ER stress-induced decreases in insulin signalling and glucose uptake suggest a critical role for this protein in muscle metabolism. Earlier studies have suggested that TRB3 may be important for glucose metabolism in skeletal muscle, although this hypothesis has not been tested directly. For example, overexpression of TRB3 in L6 cells resulted in impaired insulin signalling [9] , consistent with our data showing that TRB3 overexpression decreased insulin signalling in C2C12 cells. In another study, an acute bout of exercise decreased TRB3 expression in ob/ob mice, which the authors proposed may have contributed to the exercise-induced improvement in glucose tolerance in these animals [10] . Furthermore, muscle-specific overexpression of PGC1α in mice, which resulted in exacerbation of high-fat diet-induced insulin resistance, was associated with elevated TRB3 expression [34] . While all of these studies are consistent with TRB3 regulating glucose metabolism, our data directly tested this hypothesis through the use of multiple overexpression and knockdown models of TRB3. All of the current data demonstrate that TRB3 has an inhibitory role to decrease insulin-stimulated glucose uptake in skeletal muscle. In the current study, we detected TRB3 expression in mouse and human skeletal muscle, consistent with previous findings [6] , [10] , [34] , [35] . In contrast, in a study focused on mouse gastrocnemius muscle [33] , TRB3 protein was only shown to be expressed when the muscle underwent denervation. This is consistent with our findings, as we detected low mRNA expression of TRB3 in WG muscle ( Fig. 1a ), but observed higher expression in muscles that express oxidative red fibres, including TA, RG and Sol, suggesting that TRB3 expression may be fiber-type specific. It is interesting that denervation resulted in an increase in TRB3 expression in WG muscle [33] . As skeletal muscle denervation results in insulin resistance in this tissue [36] , [37] , [38] , it is possible that TRB3 has a role in denervation-induced insulin resistance in skeletal muscle. In addition, expression of ER stress markers has been shown to be increased in the muscle from patients with myotonic dystrophy type 1 (ref. 26 ), raising the possibility that ER stress is involved in muscle wasting-associated insulin resistance in this disease. Thus, TRB3 increases under some conditions of muscle dysfunction, and could contribute to the metabolic impairment associated with these diseases. We found that a high-fat diet in mice, and both obesity and type 2 diabetes in humans increased TRB3 expression in skeletal muscle. The mechanism by which these conditions increase TRB3 expression is not known but one possibility is that the elevated circulating insulin concentrations that are present in high-fat-fed mice and subjects with obesity and type 2 diabetes mediate the induction of TRB3 in the muscle. In support of this hypothesis, we found that insulin incubation of C2C12 myotubes for 16 h increased TRB3 expression along with increased expression of ER stress markers, which was abolished by inhibitors for PI3K and Akt. Studies in FAO hepatoma and 3T3-L1 adipocyte cells have also demonstrated that insulin induces the expression of TRB3 through C/EBPβ binding in the TRB3 promoter [39] . Taken together, these data support the hypothesis that elevated insulin concentrations could mediate the effects of high-fat feeding, obesity and type 2 diabetes to increase TRB3 expression in mouse and human skeletal muscle. Given the function of TRB3 in insulin signalling and glucose metabolism in liver [3] and β cells [8] and the increased insulin-stimulated glucose uptake in the skeletal muscle from TRB3KO mice ( Fig. 5d ), it was somewhat surprising that whole-body TRB3KO mice on a chow diet showed no alteration in glucose homoeostasis [33] . The lack of effect may be due to the different functions of TRB3 in various tissues, thereby offsetting any beneficial effects of ablation of TRB3. For example, overexpression of TRB3 in adipocytes promoted fatty acid oxidation and protected mice from high-fat diet-induced obesity [4] , whereas overexpression of TRB3 impaired glucose metabolism in liver and skeletal muscle and inhibited insulin secretion in β cells [8] . Thus, in global TRB3 knockout mice, the beneficial effects of reduced TRB3 in liver, skeletal muscle and pancreas on glucose homoeostasis may be masked by the detrimental effects of a reduction in adipocyte TRB3 expression. Although there was no change in whole-body glucose homoeostasis in TRB3 knockout mice fed a chow diet [33] , we found that TRB3 knockout mice were protected from high-fat diet-induced insulin resistance. The TRB3 knockout mice showed improved glucose tolerance, increased skeletal muscle insulin-stimulated glucose uptake and less triglyceride accumulation in the liver after 8 weeks on a high-fat diet. These data indicate that the beneficial effects of deletion of TRB3 are more pronounced under stress conditions such as high-fat feeding. It is interesting that high-fat feeding resulted in 56% lower liver triglyceride concentrations in the knockout mice, which contributed to the lower liver weights in the knockout mice. This is consistent with previous studies showing that improved insulin signalling in the liver protected mice from high-fat diet-induced hepatic steatosis, whereas impaired insulin signalling in the liver increased high-fat diet-induced lipid accumulation [40] , [41] , [42] , [43] , [44] , [45] . Thus, the lower lipid accumulation in liver of TRB3 knockout mice is presumably due to improved insulin signalling. In summary, ER stress induces expression of TRB3 in skeletal muscle, which results in impairment of insulin signalling and glucose uptake. Knockdown of TRB3 significantly blunts the effects of ER stress on glucose uptake and TRB3 knockout mice are protected from high-fat diet-induced insulin resistance. We conclude that TRB3 has an important role in ER stress-induced insulin resistance in skeletal muscle. Our data also suggest that inhibition of TRB3 expression in skeletal muscle may be a new therapeutic target for effectively managing insulin resistance. Animals Protocols for animal use and experimental procedures were conducted in accordance with NIH guidelines and approved by the Institutional Animal Care and Use Committee of the Joslin Diabetes Center. Mice were from Taconic (ICR), Charles River (C57BL/6) or were whole-body TRB3 knockout mice [33] , and were studied at 8–12 weeks of age, as specified in figure legends. Mice were maintained in a pathogen-free animal facility under standard 12-h light/12-h dark cycle, and unless indicated, were maintained on a chow diet (20% of calorie from fat; Lab Diet 5020). To study the effects of high-fat feeding, mice were fed a high-fat diet (60% of calorie from fat; Research Diets Inc D12492) beginning at the age of 6 weeks for 8 weeks. Human studies Biopsies of vastus lateralis muscle were obtained from lean (BMI=25.1±0.7 kg m −2 ), obese non-diabetic (BMI=32.6±1.5 kg m −2 ) and obese diabetic (BMI=32.8±1.1 kg m −2 ) subjects. These patients have been previously characterized [46] , and subject characteristics are presented in Supplementary Table S2 . The human studies were approved by the Institutional Review Board of the University of Texas Health Science Center at San Antonio (UTHSCSA) and the committee on human studies at the Joslin Diabetes Center (no. CHS08-22). Cell culture C2C12 myoblasts were maintained in DMEM supplemented with 10% FBS in a humidified atmosphere containing 5% CO 2 at 37 o C. When cells reached confluence in six-well plates, differentiation was induced in media containing 2% horse serum for 4 days. Adenoviruses containing TRB3 or RNAi for TRB3 were infected into the myotubes [3] , [6] , [7] . For the immunoprecipitation, 293T cells were transfected with Flag-tagged empty vector or Flag-TRB3 plasmid. Lysates were used for immunoprecipitation 2 days after the transfection. In vivo gene transfer in mouse skeletal muscle Plasmids containing Flag-tag empty vector or Flag-TRB3 were directly injected into mouse TA muscles [47] , [48] , [49] . The mice were anesthetized with an intraperitoneal injection of pentobarbital sodium (90 mg kg −1 ), and 100 μg of each DNA construct was injected longitudinally into the TA muscle with a 29-guage needle. Stainless steel electrode needles fixed 4 mm apart were then inserted into the transverse muscle belly and square-wave electrical pulses (200 V cm −1 ) were applied eight times at a rate of 1 pulse per second (duration, 20 ms) using a Grass S88 pulse generator (Grass Instruments, Quincy, MA). Our lab has demonstrated that transfection efficiency with the LacZ gene under this protocol is ~85% (ref. 47 ). Measurement of glucose uptake Muscle glucose uptake in vitro was measured [50] , [51] . Sol and EDL muscles were dissected and incubated in Krebs–Ringer bicarbonate buffer (KRB), pH 7.4, containing 2 mM pyruvate for 4 h in the presence or absence of ER stressors tunicamycin or thapsigargin. Muscles were then incubated in KRB buffer in the presence or absence of 100 nM insulin for 30 min, and glucose uptake was measured using [ 3 H]-2-deoxyglucose. Differentiated C2C12 myotubes were serum starved for 3 h in DMEM before any treatment. Cells were incubated with 100 nM insulin for 20 min. After stimulation, cells were washed with buffer containing 140 mM NaCl, 20 mM Hepes-Na (pH 7.4), 5 mM KCl, 2.5 mM MgSO 4 and 1.0 mM CaCl 2 . Glucose transport was determined by the addition of [ 3 H]-2-deoxyglucose for 10 min on ice. Cells were washed with ice-cold saline solution and harvested in 0.05 N NaOH to determine net accumulation of [ 3 H]-2-deoxyglucose [52] . RNA isolation and real-time PCR analysis Total RNA was extracted from incubated muscles or C2C12 cells using RNeasy Mini Kit (Qiagen). First-strand cDNA was synthesized using reverse transcriptase (Sigma). Primer sequences for the real-time PCR can be found in Supplementary Table S3 . Relative mRNA levels were calculated with the PCR product for each primer set normalized to TBP RNA. Western blot analysis and antibodies Tissues and cells were rapidly processed in lysis buffer [49] . Western blot analyses were used to assess protein and phosphorylation levels of various molecules. Primary antibodies purchased from commercial sources included α-tubulin, pY99, XBP1 and insulin receptor (Santa Cruz; 1:500); IRS2 (Millipore; 1:2,000); p-IRE1α (Novus Biologicals; 1:1,000); IRS1 and JNK (Upstate; 1:2,000); IRS 1Tyr 612 (Biosource; 1:2,000); and p-Akt-Thr 308 , Akt, BiP, CHOP, FoxO1, FoxO3, p-FoxO1-Ser 256 and p-FoxO3-Ser 253 (Cell Signaling; 1:2,000). Secondary antibodies used were horseradish peroxidase (HRP)-conjugated anti-rabbit (Amersham; 1:2,000), HRP-conjugated anti-mouse (Upstate; 1:3,000) and HRP-conjugated anti-goat (Promega; 1:2,000). Antibody to TRB3 was a gift from Dr Montminy [3] , [53] . Blots were developed using ECL reagents (Amersham Pharmacia) and bands were visualized and quantified using AlphaEaseFC v. 2.01 (Alpha Innotech). Statistical analysis Data are means±s.e.m. All data were compared using Student’s t -test, paired t -test, one-way analysis of variance (ANOVA) or two-way ANOVA. Correlation analyses utilized the Pearson’s coefficient. The differences between groups were considered significant when P <0.05. How to cite this article: Koh, H.-J. et al . Tribbles 3 Mediates Endoplasmic Reticulum Stress-Induced Insulin Resistance in Skeletal Muscle. Nat. Commun. 4:1871 doi: 10.1038/ncomms2851 (2013).